Observation and electric current control of a local spin in a single-molecule magnet In molecular spintronics, the spin state of a molecule may be switched on and off by changing the molecular structure. Here, we switch on and off the molecular spin of a double-decker bis(phthalocyaninato)terbium(III) complex (TbPc 2 ) adsorbed on an Au(111) surface by applying an electric current via a scanning tunnelling microscope. The d I /d V curve of the tunnelling current recorded onto a TbPc 2 molecule shows a Kondo peak, the origin of which is an unpaired spin of a π-orbital of a phthalocyaninato (Pc) ligand. By applying controlled current pulses, we could rotate the upper Pc ligand in TbPc 2 , leading to the disappearance and reappearance of the Kondo resonance. The rotation shifts the molecular frontier-orbital energies, quenching the π-electron spin. Reversible switching between two stable ligand orientations by applying a current pulse should make it possible to code information at the single-molecule level. Molecular spintronics is an emerging field of research that combines spintronics and molecular electronics [1] . Using molecules is advantageous because their electronic and magnetic properties can be manipulated under specific conditions. However, we have to have control of the spin switching and the electric-conductance variation for the realization of molecular spintronics [2] , [3] . For such a requirement, the selections of the magnetic molecule and the control mechanism of the conductance are crucial. The molecules of single-molecule magnet (SMM) are attractive, because their spin relaxation is slow and they can hold the spin information for a long time [4] . The Kondo effect has attracted attention as the conductance control mechanism, which has been observed in single atoms [5] , [6] , [7] , [8] , [9] , [10] , single molecules [11] , [12] , [13] , [14] , [15] and quantum dots [16] . The phenomenon occurs because of the interaction between conducting electrons and a localized spin [17] , and causes a change in conductance. The ability to tune the Kondo effect of SMMs would be useful for the conductance control with the use of the spin [4] , [18] . In addition, the detection of a Kondo state by using scanning tunnelling microscope (STM) should contribute to the understanding of localized spins. However, despite extensive experimental and theoretical studies [19] , [20] , little is known about the Kondo effect in SMMs. In this study, we modified the spin in a single molecule by switching on and off the localized magnetic moment of a molecular orbital. We used a double-decker bis(phthalocyaninato)terbium(III) (TbPc 2 ) molecule, which is a SMM with a high 'blocking' temperature of several tens of Kelvin, below which the relaxation of the magnetization becomes slow [21] , [22] , [23] . A spin of the molecule was detected by a clear Kondo resonance in d I /d V spectra of the tunnelling current of the STM. The Kondo effect originates from an unpaired spin in a π-orbital of the phthalocyaninato (Pc) ligands rather than from the local magnetic moment of the metal ion. We manipulated the spin by rotating the Pc ligand of a single TbPc 2 molecule by applying a current from an STM, which caused the Kondo peak to disappear. Our calculations showed that the ligand spin was quenched by a change in energy of the frontier molecular orbitals. This molecular manipulation was reversible, making it possible to switch the spin of TbPc 2 on and off as desired. In this way, we can code information in a single molecule by applying an electric current. Preparation and characterization of the adsorbed molecules TbPc 2 , which has been shown to have SMM properties, was synthesized by using a previously reported procedure with slight modifications. The complexes were deposited on a clean Au(111) surface kept at room temperature by using a sublimation method in ultra-high vacuum. The sample was then transferred to the STM head, which was cooled to ~4.7 K [24] , [25] . 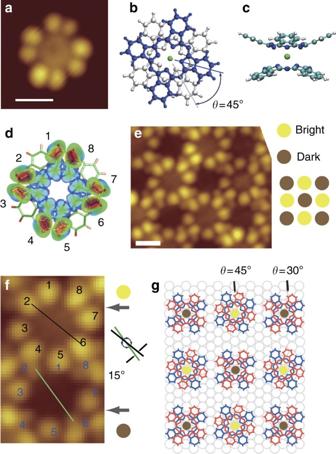Figure 1: Adsorption configuration of TbPc2on Au(111). (a) STM image of an isolated molecule of TbPc2on Au(111). (b) A schematic model of the double-decker TbPc2molecule. The upper (lower) Pc is coloured in blue (silver). (c) Side view of the TbPc2molecule after structural optimization by using DFT calculations. (d) A simulated STM image of the TbPc2molecule by DFT calculations. (e) Film of TbPc2. An alternating contrast pattern of nine molecules is shown on the right hand side with brighter molecules in yellow and darker molecules in brown. (STM images ofaandewere obtained withVsample=−0.8 V andItunnel=0.3 nA. Bars correspond to 1 nm). (f) A magnified image of bright (upper) and dark (lower) molecules. The black (green) line connects lobes 2 and 6 of bright and dark molecules. The two lines are rotated 15° with respect to each other. (g) A tentative model of the adsorption configuration of TbPc2film, corresponding to the image ine. Bright (θ=45°) and dark (θ=30°) molecules form a pseudo-square lattice, and the red and blue Pc ligands correspond to vacuum- and substrate-side Pc ligands, respectively. An STM image of an isolated TbPc 2 molecule adsorbed on Au(111) is shown in Figure 1a . The height of the molecule was determined to be ~0.40 nm, and eight bright lobes were visible at the perimeter of the molecule. To explain the image, we developed a model and simulated an STM image for TbPc 2 adsorbed on Au(111) surface. In TbPc 2 , two Pc ligands sandwich a Tb ion. Figure 1b shows a top view of the molecule, in which upper and lower Pc ligands are coloured in blue and silver, respectively, with an azimuthal rotational angle ( θ ) between the two Pc ligands of 45°. The two Pc ligands adopt a bent configuration with respect to each other, as shown in Figure 1c . Figure 1: Adsorption configuration of TbPc 2 on Au(111). ( a ) STM image of an isolated molecule of TbPc 2 on Au(111). ( b ) A schematic model of the double-decker TbPc 2 molecule. The upper (lower) Pc is coloured in blue (silver). ( c ) Side view of the TbPc 2 molecule after structural optimization by using DFT calculations. ( d ) A simulated STM image of the TbPc 2 molecule by DFT calculations. ( e ) Film of TbPc 2 . An alternating contrast pattern of nine molecules is shown on the right hand side with brighter molecules in yellow and darker molecules in brown. (STM images of a and e were obtained with V sample =−0.8 V and I tunnel =0.3 nA. Bars correspond to 1 nm). ( f ) A magnified image of bright (upper) and dark (lower) molecules. The black (green) line connects lobes 2 and 6 of bright and dark molecules. The two lines are rotated 15° with respect to each other. ( g ) A tentative model of the adsorption configuration of TbPc 2 film, corresponding to the image in e . Bright ( θ =45°) and dark ( θ =30°) molecules form a pseudo-square lattice, and the red and blue Pc ligands correspond to vacuum- and substrate-side Pc ligands, respectively. Full size image Structures of TbPc 2 adsorbed on Au(111) surface were elucidated using density functional theory (DFT). A simulated STM image of the TbPc 2 molecule on Au(111) is shown in Figure 1d . The eight protrusions in the simulated STM image are from the upper Pc ligand. The lower Pc ligand does not contribute directly to the image. An STM image of a monolayer film of TbPc 2 molecules obtained with a sample bias ( V sample ) of −0.8 V is shown in Figure 1e . Nine full molecules, which make a pseudo-square lattice, were visible in the image. The image showed a checkerboard contrast pattern, which is depicted on the right hand side of Figure 1e . The bright molecules (b) and the dark molecules (d) are shown in yellow and brown, respectively. Magnified images of two neighbouring molecules are shown in Figure 1f , in which the top and bottom molecules correspond to b and d, respectively. Eight lobes were clearly observed for b, which are marked as 1–8. However, in the image of d, we observed four tiny lobes (marked 2, 4, 6 and 8), and the four other lobes (1, 3, 5 and 7) were either shadowed or shared by bright lobes of the neighbouring b. The b and d molecules were rotated with respect to each other, which can be clarified by drawing lines connecting the bright lobes. Lobes 2 and 6 or 4 and 8 were used because they were clearly observed for both b and d. The lines connecting lobes 2 and 6 of b and d were rotated by 15° with respect to each other. As described in the Methods section, the bottom Pc ligand of each molecule was aligned in the same direction, and the upper Pc ligand was aligned such that θ ≈45° for b and 30° for d (see Fig. 1g ). The values of θ alternate because of the steric repulsion between the upper Pc ligands. If θ ≈45° for every molecule, the phenyl rings would interfere with each other. 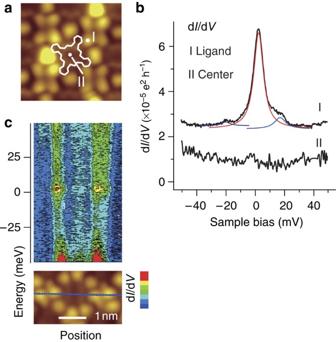Figure 2: STS measurement of TbPc2near Fermi level. (a) STS detection positions on the film together with a model of the upper Pc plane. (b) dI/dVspectra at I and II ina. (c) Change in the Kondo peak height when the tip position was moved along the blue line in the STM topography panel. The different colours correspond to the dI/dVintensity, described below the figure. Kondo resonance detected by tunnelling spectroscopy Figure 2 shows the analysis of tunnelling conductance (d I /d V ) on a TbPc 2 molecule. The zero-bias peak (ZBP) was assigned to a Kondo resonance. We observed clear Kondo features for the molecules with θ ≈45° when the tip was positioned over one of the lobes of b (labelled I in Fig. 2a,b ). However, when the tip was placed over the centre of the molecule, only a small feature was observed (mark II in Fig. 2a,b ). A sample temperature of 4.3 K and a modulation voltage of 1 mV, corresponding to an estimated resolution of 3 meV [26] were used. Figure 2: STS measurement of TbPc 2 near Fermi level. ( a ) STS detection positions on the film together with a model of the upper Pc plane. ( b ) d I /d V spectra at I and II in a . ( c ) Change in the Kondo peak height when the tip position was moved along the blue line in the STM topography panel. The different colours correspond to the d I /d V intensity, described below the figure. Full size image In Figure 2b , spectrum I was obtained by subtracting a smooth background. In the spectra shown hereafter, the conductance of the background curve at the Fermi level (zero bias) was calibrated to 1.2×10 −9 (A/V), which is equivalent to 3.2×10 −5 (e 2 h −1 ). We observed a large ZBP and two small side peaks, which were fitted as shown in spectrum I. Figure 2c shows the changes in the d I /d V spectra near the Fermi level (upper panel) as the tip was moved along the symmetry line of TbPc 2 shown in the lower panel. A Kondo peak was observed only when the tip was positioned over the bright spots, and no peak was observed when the tip was over the centre of the ligand. The site dependence of the Kondo peak is different from previous reports involving metal–Pc complexes, such as FePc and CoPc, which only show a Kondo peak when the tunnelling electrons are injected in the centre of the molecule [11] , [12] , [27] . This suggests that the mechanism for the appearance of the Kondo resonance in TbPc 2 is different from that for MPc, and that the Pc ligand and its spin have an important role in the TbPc 2 case. To prove that the Kondo resonance is the origin of the ZBP, we examined the changes in the peak width and height in relation to both the sample temperature and the presence of a magnetic field. 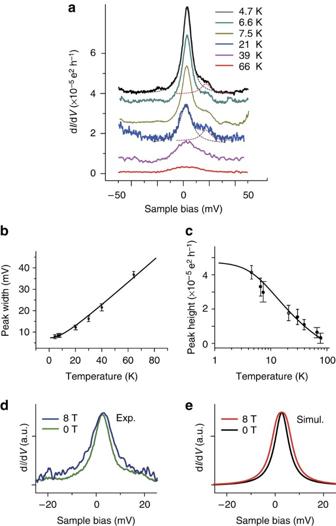Figure 3: Proving the assignment of the ZBP to the Kondo feature. (a) Temperature dependence of the peaks measured in the region of 4.7–66 K. Background curves were subtracted. (b,c) Peak width (b) and peak height (c) changes versus temperature for the peak near the Fermi level. The dotted curves indicate the fitted curves mentioned in the text. The error bars correspond to the distribution of the measured data of more than ten samplings. (d,e) Peak changes in the presence of a magnetic field of 8 T;dis experimental (exp.) data andeis a simulation (simul.) of two convoluted peaks separated by two times the Zeeman splitting for the Kondo effect (see text). The dependence on the temperature is shown in Figure 3a , with fitted curves for T =4.7 K and 21 K superimposed as dotted lines. The ZBP broadened, and the height decreased as the temperature increased, as shown in Figure 3b,c . Figure 3: Proving the assignment of the ZBP to the Kondo feature. ( a ) Temperature dependence of the peaks measured in the region of 4.7–66 K. Background curves were subtracted. ( b , c ) Peak width ( b ) and peak height ( c ) changes versus temperature for the peak near the Fermi level. The dotted curves indicate the fitted curves mentioned in the text. The error bars correspond to the distribution of the measured data of more than ten samplings. ( d , e ) Peak changes in the presence of a magnetic field of 8 T; d is experimental (exp.) data and e is a simulation (simul.) of two convoluted peaks separated by two times the Zeeman splitting for the Kondo effect (see text). Full size image Nagaoka et al . [28] introduced a formula for the temperature dependence of the Kondo-peak width on temperature ( Γ ( T )) using Fermi-liquid theory: where k B is the Boltzmann constant and T K is the Kondo temperature. The observed data (solid circles) were fitted using this formula, and the fitted curve is shown in Figure 3b as a solid line. T K was determined to be ~31 K. This temperature is very low compared with other reported values: T K >200 K for CoPc [11] , T K =357 and 598 K for FePc with different bonding configurations [27] , and T K =105 and 170 K for different conformations of TBrPP-Co [12] . Furthermore, the decrease in height of ZBP with an increase in the temperature is the evidence for a Kondo resonance. An empirical relation for the temperature dependence of the Kondo-induced conductance, G , was used to characterize the Kondo resonance [29] : G ( T )= G 0 ( T ′ 2 K / T 2 + T ′ 2 K )s, where G 0 is the G value at zero temperature and . Thus, G ( T K )is equal to G 0 /2. The decay behaviour observed in Figure 3c could be reproduced using a T K of 31 K and an empirical parameter s of 0.2. The behaviour of ZBP in relation to an applied magnetic field was studied. The Kondo resonance splits when a magnetic field was applied, and this splitting is two times larger than the ordinary Zeeman splitting [30] . Figure 3d shows a comparison of the d I /d V spectra in magnetic fields of B =0 and 8 T. When B=8 T, the spectrum is broader by ~2 meV. Although clear splitting of the Kondo peak in the presence of the magnetic field has been reported previously [31] , it was not clear in Figure 3d . We simulated the changes in the peak by convoluting two Lorentzian peaks with Γ =6.5 meV and separated by 1.8 meV (two times the Zeeman splitting energy at 8 T) around the Fermi level into a single peak (see Fig. 3e ). Because of the original peak width when B =0 T, the splitting was not obvious except for a slight broadening of ~1 meV. This simulation supports our assignment of the peak to be a Kondo resonance. 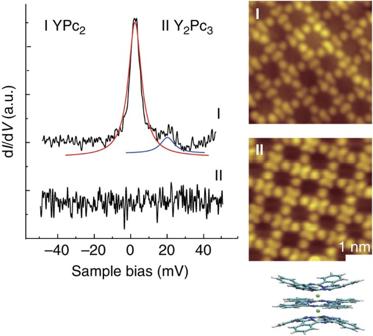Figure 4: Kondo peaks in related molecules. Comparison of the dI/dVcurves for I YPc2and II Y2Pc3. Corresponding STM images are shown in the right hand side (Vsample=0.8 V andItunnel=0.3 nA). A side view of Y2Pc3is superimposed. To further investigate the mechanism of the appearance of the Kondo feature, we acquired d I /d V spectra of double-decker YPc 2 and triple-decker Y 2 Pc 3 , as shown in Figure 4 . We prepared the non-SMM double-decker complex YPc 2 and the non-SMM triple-decker complex Y 2 Pc 3 [32] . A sharp Kondo feature appeared for YPc 2 , whereas there was no Kondo peak for Y 2 Pc 3 . Below, we discuss the mechanism of the presence/absence of the Kondo feature in terms of the spins of the metal atoms and the electronic configuration of the ligands. Figure 4: Kondo peaks in related molecules. Comparison of the d I /d V curves for I YPc 2 and II Y 2 Pc 3 . Corresponding STM images are shown in the right hand side ( V sample =0.8 V and I tunnel =0.3 nA). A side view of Y 2 Pc 3 is superimposed. Full size image Spin control by molecular structure manipulation The configuration of the π-electrons has an important role in the appearance of Kondo peaks, and its manipulation should make it possible to control Kondo states. To determine if this is possible, we rotated the upper Pc ligand by injecting enough current via the STM tip to overcome the activation barrier for the conformation change. 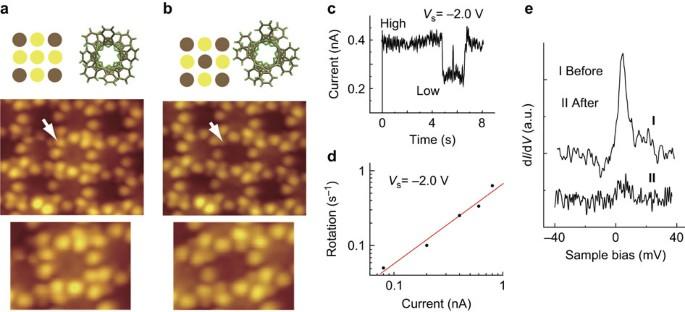Figure 5: Molecular manipulation and control of Kondo feature. (a,b) Conversion of the centre molecule from b (θ=45°) to d (θ=30°) by applying a current pulse. The target molecule is marked by an arrow, and magnified images are shown in the bottom panel. Changes in the contrast and the top view of the centre molecule are schematically illustrated. (c) Current during a −2.0 V voltage pulse over a TbPc2molecule initially in the b state; the tip remained fixed over a lobe position with the feedback loop open. Each jump in the current indicates the moment of rotation of the molecule and the low state corresponds to the d state. (d) Rotations per electron as a function of tunnelling current forV=−2.0 V. Both axes are in log scale. More than 50 molecules similar to the one inawere sampled. Data shown are for rotation from b to d. The red line corresponds to a least squares fit. (e) Comparison of the Kondo peaks before I and after II the application of the pulse. Figure 5a,b shows an STM image, in which the centre molecule was converted from b ( Fig. 5a ) to d ( Fig. 5b ) by applying a pulse V sample to the molecule. We believe that the lower Pc ligand does not move, and rotation of the upper Pc ligand changes θ . Figure 5: Molecular manipulation and control of Kondo feature. ( a , b ) Conversion of the centre molecule from b ( θ =45°) to d ( θ =30°) by applying a current pulse. The target molecule is marked by an arrow, and magnified images are shown in the bottom panel. Changes in the contrast and the top view of the centre molecule are schematically illustrated. ( c ) Current during a −2.0 V voltage pulse over a TbPc 2 molecule initially in the b state; the tip remained fixed over a lobe position with the feedback loop open. Each jump in the current indicates the moment of rotation of the molecule and the low state corresponds to the d state. ( d ) Rotations per electron as a function of tunnelling current for V =−2.0 V. Both axes are in log scale. More than 50 molecules similar to the one in a were sampled. Data shown are for rotation from b to d. The red line corresponds to a least squares fit. ( e ) Comparison of the Kondo peaks before I and after II the application of the pulse. Full size image Rotation of a molecule can be monitored by the tunnelling current change, helping to understand the mechanism of the rotation. Figure 5c shows changes in the current during injection of a current pulse with V sample =−2.0 V. The high and low states of the tunnelling current correspond to b and d, respectively. The sharp changes in the current indicate when rotation occurs. We rotated the upper Pc ligand of more than 50 molecules and obtained an average rate [33] of rotation ( R ) from b to d as a function of the current ( I ). The results are summarized in Figure 5d for V sample =−2.0 V. Least squares analysis of a plot of log( R ) versus log( I ) yielded a slope of ~1.09. Thus, the reaction order n in the relation R I n should be close to 1. This suggests that the current-induced rotation is a one-electron phenomenon. Various surface manipulations have been performed with a similar mechanism [34] . In the present case, the injected electron provided enough energy to turn the upper Pc ligand. Once the molecule switches to the other state by the pulse current, it stays there for hours, allowing us to image and characterize the new conformation in subsequent STM studies. The Kondo peaks, which were obtained at the bright spots, dramatically changed after the application of the pulse, as shown in Figure 5e . In fact, the sharp Kondo feature disappeared when d formed (see for example Fig. 5b ). Our data show that an unpaired electron in a π-orbital of the upper Pc ligand is responsible for the appearance of the Kondo peak for TbPc 2 . As TbPc 2 is neutral, there must be a +1 π-radical because the molecule is composed of a Tb +3 ion and two Pc −2 ligands (totally −4) [23] . Thus, one of the ligands should have an unpaired electron in a π-orbital [35] . The correlation between the appearance of the Kondo peak and the presence of an unpaired electron in a π-orbital can be seen more clearly in the comparison between double-decker YPc 2 and triple-decker Y 2 Pc 3 (see Fig. 4 ). Both molecules contain a Y ion in a +3 oxidation state. Thus, in the double-decker complex, there is a single unpaired electron in the π-orbital of the Pc ligand and no spin on the Y ion. In the triple-decker molecule, the two Y ions have a total oxidation state of +6 with no d or f spin, and the sum of the oxidation states of the three Pc ligands is −6, which means that Y 2 Pc 3 is neutral and has no spin system. We observed a sharp Kondo feature for YPc 2 , whereas no Kondo peak was observed for Y 2 Pc 3 . In other words, the Kondo feature occurs because of an unpaired π-electron in a ligand orbital instead of a metal orbital. The Kondo state is formed in the presence of degenerate spin states. In the case of TbPc 2 , there are two spin systems: one spin system involves the central Tb ion (4f electrons, J = L + S =±6) and the other involves one unpaired electron in a π-orbital. In the present case, the large magnetic anisotropy on the Tb ion leads to a loss of the spin degeneracy and effectively hampers the formation of a Kondo state. However, the two degenerate spin states ( S =1/2) of the π-electron together with its sizable coupling to the substrate lead to the measurable Kondo peak mentioned above. We demonstrated that the Kondo feature can be switched on and off by changing θ , as shown in Figure 5 . To understand the change in the Kondo resonance with respect to θ , we examined the changes in the π-orbitals in relation to θ by using spin-resolved DFT calculations. When θ =45°, the Pc ligand of the molecule on a Au(111) surface had an S =1/2 spin. Vitali et al . have reported similar calculations [35] . However, they only observed a spin in the π-orbitals of isolated molecules and none in those of molecules adsorbed on a Cu(111) surface. This is due to charge transfer from the Cu surface to the molecule, causing the electron in the π-orbitals of the ligand to pair up. In our case, TbPc 2 does not interact strongly with the Au(111) surface leading to a smaller degree of charge transfer. In other words, an unpaired spin remains in the π-orbitals after adsorption. It is important to determine the spatial distribution of the unpaired π-electron both in the fundamental understanding of the Kondo resonance and in the control of the spin. However, it is not easy to do solely by the STM measurement. Alternatively, we visualized the spin polarization by calculating the difference of the density of the up-spin and the down-spin (see Supplementary Fig. S1 ). The result indicates that the higher spin-polarization sites are accumulated only in the upper Pc. This is because, upon adsorption on the Au surface, the upper and lower Pc are not equivalent, which is the effect of the metallic surface to create a dipole that localizes the electronic charge in the molecule. As the upper Pc plane rotates from θ =45°, the energy levels of both the singly occupied molecular orbital (SOMO) and the highest occupied molecular orbital (HOMO) change. 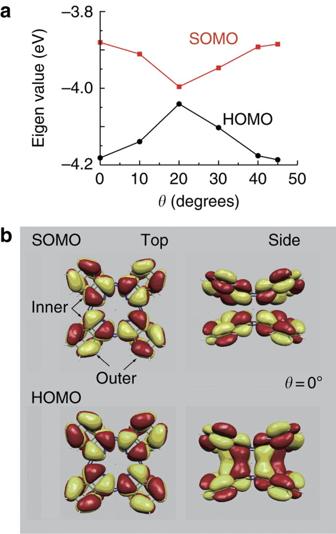Figure 6: Energy level and level crossing of SOMO and HOMO. (a) Change in the peak positions of the SOMO and HOMO levels versusθdetermined by using DFT calculations. (b) Molecular orbitals for SOMO and HOMO forθ=0° Top view shows eight lobes both for outer circles and inner circles of the molecule. In the side view, a bonding between the two Pc can be seen in HOMO. Note the phase difference of the upper and lower Pc of SOMO and HOMO. We computed these changes for an isolated molecule, and the peak positions of the SOMO and HOMO levels for the minority spin are plotted in Figure 6a . As θ changed from 45°, the SOMO and HOMO levels became closer in energy. This can be clearly understood if we consider the level crossing of the two levels. We calculated molecular orbitals for SOMO and HOMO for θ =0° (see Fig. 6b ). The difference in SOMO and HOMO is the phase in the upper and lower Pc ligand; they are in-phase for HOMO and 180 ° anti-phase for SOMO, which can be clearly seen by the bonding between the two Pc in the inner circle of the HOMO states. This is reasonable because the HOMO state should be energetically more stable than the SOMO state. The bonding is mainly formed in the inner circle, which is due to the bent configuration of the molecule that makes the distance between the upper and lower lobes of the inner circles smaller than that of the outer. When we rotated by 45°, the lobes in the inner circles change their phase completely. They become in-phase for SOMO state and anti-phase for HOMO state. According to the definition that the HOMO is more stable than the SOMO, the HOMO state at θ =0° now becomes SOMO at θ =45°. This is how the level crossing occurs at θ between 0° and 45°. Figure 6: Energy level and level crossing of SOMO and HOMO. ( a ) Change in the peak positions of the SOMO and HOMO levels versus θ determined by using DFT calculations. ( b ) Molecular orbitals for SOMO and HOMO for θ =0° Top view shows eight lobes both for outer circles and inner circles of the molecule. In the side view, a bonding between the two Pc can be seen in HOMO. Note the phase difference of the upper and lower Pc of SOMO and HOMO. Full size image Finally, in the presence of the Au(111) surface, the SOMO became doubly occupied near θ =30° due to charge transfer from the surface, quenching the molecular spin and hence the Kondo state. In conclusion, by using controlled current pulses, we rotated the upper Pc ligand in TbPc 2 , which led to the disappearance of the π-orbital spin. This is due to charge transfer from the substrate to the SOMO level, as the SOMO level decreases in energy, approaching the Fermi energy, upon ligand rotation. The π-orbital spin, which is localized on the upper ligand, appeared as a Kondo peak in electronic conductance spectra. The large magnetic moment of the metal ion does not produce a Kondo signal because the intrinsic molecular anisotropy impedes the formation of a degenerate state needed for the Kondo spin flip to occur. Hence, TbPc 2 on Au(111) is a spin one-half Kondo system because of the ligand spin. The upper ligand could be rotated in a controlled manner, switching on and off the spin. Thus, information can be encoded on the single-molecule level by controlling the molecular spin via an electric current. Synthesis of double- and triple-decker molecules All reagents were purchased from Wako or Aldrich and used without further purification. The compounds were prepared following reported procedures with slight modifications [21] , [36] . A mixture of 1,2-dicyanobenzene (62.7 mmol), M(OAc) 3 ·4H 2 O (M=Tb, Dy and Y; 3.92 mmol) and 1,8-diazabicyclo[5,4,0]undec-7-ene (33.5 mmol) in 200 ml of 1-hexanol was refluxed for 1.5 days. The solution was allowed to cool to room temperature and then filtered. The precipitate was washed with acetic anhydride, cold acetone and n -pentane. Then, the precipitate was dried in air. The crude purple product was extracted with ten 200 ml portions of CHCl 3 . The green extracts were combined and concentrated, and column chromatography (C-200 silica gel, Wako) was used to isolate the product with 98:2 CH 2 Cl 2 /MeOH as the eluent. The green fraction, which was also the first fraction, was collected while being careful not to contaminate with the fraction containing the [MPc 2 ] −1 complex, which was the second fraction (blue-green). The green fraction was concentrated, and n -hexane was added until the compound got precipitated. The green precipitate was filtered and dried in vacuo . In general, the yield was 2–5%. Preparation of substrate and molecule deposition The substrate was a single crystal Au(111) surface, which was prepared in a ultra high vacuum by repeated sputtering with Ar + and annealing at 900 K. The molecule was deposited on the Au(111) surface by evaporation from a Ta boat after prolonged degassing. X-ray photoemission spectroscopy was performed using non-monochromatized X-ray source of Al Kα (XSAM 800pci, Kratos) to check the composition of the deposited molecules. TbPc 2 , YPc 2 and Y 2 Pc 3 were deposited at a flux rate of ~0.1 monolayer per minute, with the Au substrate at room temperature. No subsequent annealing was executed after the deposition. The substrate cleaning, molecule deposition and low-temperature STM observations were done in ultra high vacuum chambers connected by metal valves. The sample could be transferred between them without exposure to air. The STM head was placed in a tube-like stainless chamber, which was inserted into a He dewar. The He dewar was attached to an air-suspended table and was located below floor level. The assembly comprised of the tube scanner, STM tip and sample holder, and inertia slider for coarse motion of the tip was suspended by springs to isolate it from vibration. Scanning tunneling spectroscopy (STS) spectra were obtained using a lock-in amplifier in which a modulation voltage of 1 mV was superimposed onto the tunnelling bias voltage. Model of the TbPc 2 film and configuration of TbPc 2 molecule The lattice of the TbPc 2 film can be expressed with the two vectors of b1 and b2 (see Supplementary Fig. S2 ), in which b1 is parallel to with a length of 5 a ( a is the nearest neighbour distance of Au atoms, a ~0.288 nm) and b2 is parallel to with a length of . Similar structures have been reported for FePc [27] and CoPc [37] molecules adsorbed on the Au(111) surface. We assume that the bonding configuration of the bottom Pc is same as that of the FePc [27] and CoPc [37] molecules adsorbed on the Au(111) surface, in which the azimuthal rotation is aligned such that the line connecting the centres of the diagonal phenyl rings is parallel to the direction, which is rotated 60° from the direction (see Supplementary Fig. S2 ). Furthermore, we consider the azimuthal rotation of the upper and lower Pc of each TbPc 2 molecule. In our model (see Supplementary Fig. S3a ), the upper Pc (red) is rotated 45° with respect to the lower Pc (blue). We chose this twist angle as it is close to the angle observed in the bulk crystal (~42°). As the lower Pc is aligned in the direction, the symmetry line connecting the two phenyl groups of the upper Pc, s, makes an angle of φ =75° from the vertical line, v. We calculated the distribution of HOMO orbital by Vienna ab-initio simulation program (VASP) (see Supplementary Fig. S3b ). The symmetry line of s defined in Supplementary Figure S3a is also illustrated. In Supplementary Figure S3c , the bright (upper) and dark (lower) molecules were magnified in the STM image. The two molecules are aligned in the direction and are placed parallel to the vertical direction of the figure. In a similar manner as shown in Supplementary Figure S3b , we draw the symmetry line s for the bright molecule. The measured angle between s and v was ~75°, which coincides with the model of Supplementary Figure S3a . Thus, we believe that the assumption of the azimuthal angle of lower Pc and the rotation angle of 45° of the upper Pc can reproduce the distribution of the observed lobes of the TbPc 2 molecules well. The rotation of angle of the dark molecule was explained in the main manuscript. HOMO state STS spectra of TbPc 2 We showed an example of the change of the HOMO and SOMO energy with the rotation of the azimuthal angle of the upper and lower Pc in the Figure 6 , change of which was ~0.1 eV. We further claimed that the molecular spin is altered because the number of electrons that occupy the SOMO state changes. One of the conditions required for this discussion is that the state is sharp enough such that the energy level change of ~0.1 eV can significantly modify the number of the electrons occupied in the state. To see whether the electronic states of the molecule satisfy this condition, we measured STS spectra obtained on the molecule (see Supplementary Fig. S4 ). We see a sharp peak at the energy of ~100 meV in the occupied state, and the full-width at half-maximum of the peak is ~40 meV. This indicates that the broadening of the molecule's electronic state is limited, and the ~0.1 eV change in the electronic state should have a meaningful change for the electron-occupancy of the molecule. DFT calculation First-principle calculations were performed by using VASP code, employing a plane wave basis set and projector augmented wave (PAW) potentials to describe the behaviour of valence electrons [38] , [39] . A generalized gradient Perdew Burke Ernzerhof exchange-correlation potential [40] was used. The structures were relaxed until the forces were smaller than 0.05 eV Å −1 . Because of the absence of dispersion forces in the local and semilocal exchange-correlation approximations, the molecule-surface distance was only an estimate. Therefore, little can be said on the charge transfer from the substrate to the molecule. As first approximation, free molecules were used to discuss the electronic structure. However, the simulations of the STM images included the gold surface, which was modelled as a five-atom-thick slab, and were based on the lateral arrangement of TbPc 2 molecules described in the results. The Tersoff and Hamman theory [41] was used to compute the STM images using a previously reported method [42] . How to cite this article: Komeda, T. et al . Observation and electric current control of a local spin in a single-molecule magnet. Nat. Commun. 2:217 doi: 10.1038/ncomms1210 (2011).